Composite pulses for robust universal control of singlet–triplet qubits Precise qubit manipulation is fundamental to quantum computing, yet experimental systems generally have stray coupling between the qubit and the environment, which hinders the necessary high-precision control. Here, we report the first theoretical progress in correcting an important class of errors stemming from fluctuations in the magnetic field gradient, in the context of the singlet–triplet spin qubit in a semiconductor double quantum dot. These errors are not amenable to correction via control techniques developed in other contexts, as here the experimenter has precise control only over the rotation rate about the z axis of the Bloch sphere, and this rate is furthermore restricted to be positive and bounded. Despite these strong constraints, we construct simple electrical pulse sequences that, for small gradients, carry out z axis rotations while cancelling errors up to the sixth order in gradient fluctuations, and for large gradients, carry out arbitrary rotations while cancelling the leading order error. A quantum computer would permit exponentially faster algorithms than an ordinary computer for certain important types of problems [1] . Universal quantum computation requires the ability to perform an entangling two-qubit gate and precise single-qubit rotations around two different axes of the Bloch sphere. Single-electron spin qubits in semiconductor quantum dots potentially have marked advantages in fast two-qubit gating and scalability [2] , but suffer an embarrassing difficulty in performing fast single-qubit rotations because the strong, high-frequency magnetic fields naïvely required [3] heat the sample and are hard to confine to a single qubit [4] . This problem is circumvented by encoding the qubit in the low-lying singlet–triplet subspace of a two-electron double quantum dot [5] , [6] , [7] , [8] . Fast electrical control of the exchange coupling, J , via the tilt of the effective double-well potential allows sub-ns rotations about the z axis of the Bloch sphere. To perform arbitrary rotations of such a qubit, though, one must introduce a difference, ΔB , between the local magnetic fields at each dot, resulting in rotation about the x axis of the Bloch sphere. This can be done either by pumping a nuclear spin polarization gradient [9] or by depositing a micromagnet nearby [10] . However, a problem remains: the local magnetic field typically fluctuates slowly due to second-order nuclear spin flip-flops mediated by the hyperfine coupling to the electron spin [11] , [12] and owing to charge-noise-induced shifts of the double-dot position in the inhomogeneous field. The resulting uncertainty in ΔB introduces a quasi-static random component to the rotation about the x axis that, in the course of ensemble averaging, leads to rapid decoherence of the qubit on the free induction decay timescale of T 2 * . However, the fact that these errors implement coherent rotations (albeit by an unknown angle) makes it possible to reduce their effect by means of dynamical control; this nice feature is due to the non-Markovian nature of the nuclear spin bath, a situation unique to quantum dot spin qubits. In the case of quantum memory, dynamical decoupling techniques [7] , [12] , [13] , [14] , [15] , [16] , [17] can be employed to preserve qubit information long beyond T 2 * , up to a timescale T 2 (which is defined with respect to a specific dynamical decoupling sequence) at which this information is ultimately lost due to dynamical fluctuations. This ability is crucial, because typically T 2 10 4 T 2 * for localized electron spins in semiconductors—in particular, in GaAs quantum dot systems [6] , [7] , T 2 * ~ 10 ns, T 2 ~0.1 ms, and in Si [8] , T 2 * ~ 100 ns with T 2 predicted [18] to be ~1 ms. However, such echo techniques cannot be performed simultaneously with arbitrary single-qubit rotations, so gate errors are still dominated by statistical fluctuations and depend on the ratio of the gate time to T 2 * rather than to T 2 . It is of utmost importance to address this problem because fault-tolerant quantum computation requires extremely precise single-qubit rotations. Thus, the task is to find dynamically corrected gates [19] , [20] , [21] , [22] , [23] applicable to singlet–triplet qubits. Finding such gates is challenging because available control in real experimental singlet–triplet spin qubit systems is rather limited: One only has precise control over the rotation rate about the z axis of the Bloch sphere via the exchange interaction, and because of the nature of the exchange interaction, this rotation rate is intrinsically restricted to be positive and bounded. Meanwhile, the rotation around the x axis due to the magnetic field gradient cannot be precisely controlled. These control constraints specific to singlet–triplet qubits render the numerous quantum control techniques developed in other fields, such as nuclear magnetic resonance, inapplicable. In this work, we show how to perform dynamically corrected single-qubit gates on singlet–triplet qubits, dramatically reducing errors while fully respecting these experimental constraints. We construct simple electrical pulse sequences that, for small magnetic field gradients, carry out rotations about the z axis while cancelling gate errors up to the sixth order in the gradient fluctuations, and for large magnetic field gradients, carry out arbitrary rotations while cancelling the leading order error. This represents an important step forward in the development of singlet–triplet qubits as viable resources for quantum computing. Model We consider the Hamiltonian governing the singlet–triplet qubit, with constraints on the parameters imposed to account for the physical realities of the experiments [6] , [7] , [8] , [9] , [17] , [24] , [25] . Here h = gμ B ΔB and fluctuations in ΔB are much slower than typical gate times so that h = h 0 + δh with h 0 a known constant and δh a random, unknown constant. ( T 2 * is inversely proportional to the width of the statistical distribution from which δh is drawn. We estimate the effect of high-frequency noise components in the Supplementary Discussion .) The qubit is manipulated via the electrically controlled exchange coupling, J ( t ), which is constrained to be positive (except in very high magnetic fields, when it is always negative) and is restricted in magnitude either by the practice of keeping the qubit near the zero-bias point to reduce charge noise sensitivity, or, more intrinsically, by the singlet–triplet splitting of two electrons on a single dot, so that 0 J ( t ) J max . The constraint to positive rotations is also relevant to exchange-only coded qubits [26] , [27] , [28] . Our goal is to design a pulse in J ( t ) that respects these constraints and performs a given rotation in a way that is insensitive to δh . We dub the resulting composite pulse sequence SUPCODE: soft uniaxial positive control for orthogonal drift error. We emphasize that although the singlet–triplet qubit is one of the most experimentally advanced paths towards a scalable quantum computer, the restricted control available does not permit application of existing elegant methods of quantum control. In particular, the positivity of J ( t ) precludes the prescriptions of refs 19 , 20 (which anyway do not accommodate universal single-qubit operations) and ref. 21 . Although other works allow a positivity constraint [22] , [23] , they are nonetheless precluded by the uncontrolled, always-on gradient h . Below we consider two cases: h 0 =0, which is directly relevant to experiments with unpumped nuclear spins and no micromagnet [6] , [8] , where only rotations about the z axis are desired (for example, for spin echo), and h 0 ~ J max , which is directly relevant to experiments with pumped nuclear spins [9] or a nearby micromagnet [10] where full single-qubit control is desired. SUPCODE for h 0 =0 For h 0 =0, we assume for simplicity that the pulse is of a binary form where J ( t ) alternates between its extremal values of 0 and J max . Expanding the evolution operator of the system, , in powers of δh / J max , we choose the time duration of each segment such that the zeroth order term is a rotation about by the desired angle and one or more successively higher order terms vanish. We give details in the Methods, and in Supplementary Discussion, we also rigorously show that there is no pulse that cancels all higher orders for finite J max . Thus, we find three-, five-, seven-, and nine-piece SUPCODE pulses that perform arbitrary rotations about while cancelling undesired terms up to the first, second, second, and third order in δh / J max , respectively. (We note that in this special case, the first order cancellation could also be performed via ref. 23 .) An example of the five-piece SUPCODE pulse, which cancels first and second order terms in δh / J max in the evolution operator (corresponding to second and fourth order terms in the gate error), is shown in Fig. 1 . Figure 2 traces the evolution of a particular initial state on the Bloch sphere under a five-piece SUPCODE pulse designed to perform a π /2 rotation about . 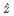Figure 2: Example of evolution of a given state on the Bloch sphere under the five-piece SUPCODE, rotating aroundbyπ/2 . Hereh0=0, and for the purpose of illustration, we have takenδh/Jmax=0.05.labels the state with the spin-up (spin-down) electron occupying the left (right) dot. Likewise,labels the spin-permuted state.denotes the singlet statedenotes the non-magnetic triplet state. The green arrow is the Bloch vector pointing to the final state after the evolution, which is represented as a point on the surface of the Bloch sphere. The black curve shows the trajectory of the state under the five-piece SUPCODE. 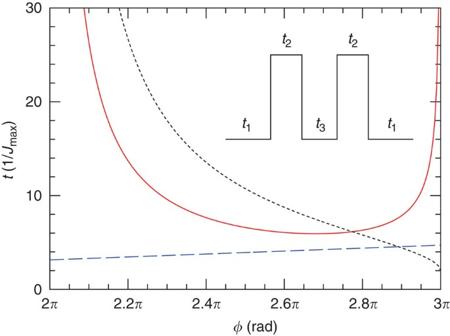We include an animation showing how this state evolves under the five-piece SUPCODE pulse in Supplementary Movie 1 . Figure 1: Example of the five-piece SUPCODE pulse cancelling gate error up to the fourth order inδhforh0=0. The inset shows a schematic profile of such a pulse as a function of time. The time duration of each piece is denoted byt1,t2, andt3. In the main panel, we show the values oft1(red solid line),t2(blue dashed line), andt3(black dotted line) as functions of the rotation angleφ. Figure 1: Example of the five-piece SUPCODE pulse cancelling gate error up to the fourth order in δh for h 0 =0. The inset shows a schematic profile of such a pulse as a function of time. The time duration of each piece is denoted by t 1 , t 2 , and t 3 . In the main panel, we show the values of t 1 (red solid line), t 2 (blue dashed line), and t 3 (black dotted line) as functions of the rotation angle φ . Full size image Figure 2: Example of evolution of a given state on the Bloch sphere under the five-piece SUPCODE, rotating around by π /2 . Here h 0 =0, and for the purpose of illustration, we have taken δh / J max =0.05. labels the state with the spin-up (spin-down) electron occupying the left (right) dot. Likewise, labels the spin-permuted state. denotes the singlet state denotes the non-magnetic triplet state . The green arrow is the Bloch vector pointing to the final state after the evolution, which is represented as a point on the surface of the Bloch sphere. The black curve shows the trajectory of the state under the five-piece SUPCODE. Full size image We define the average error per gate, Δ, as where V is the desired operation, U ( T f ) is the actual evolution operator under the composite pulse of duration T f , and the overlap is averaged over initial states | ψi > distributed uniformly over the Bloch sphere. Fig. 3 shows the average error per gate for the naïve one-piece pulse and the SUPCODE pulses introduced above. We see that for δh / J max <10% the SUPCODE pulses have markedly less error. This range is relevant to recent landmark experiments with GaAs [7] and silicon-based [8] double quantum dots. In the former δh ~8 neV and in the latter δh ~3 neV, while in both cases J max could be several hundred neV. We also see that although the leading order of the error for the nine-piece pulse is higher than that of the other pulses, its coefficient is large enough that for δh / J max 2%, it is better to use the five- or seven-piece pulses. This suggests that generating similar pulses with even more pieces likely will not extend the range of values of δh for which low-error rotations are possible. 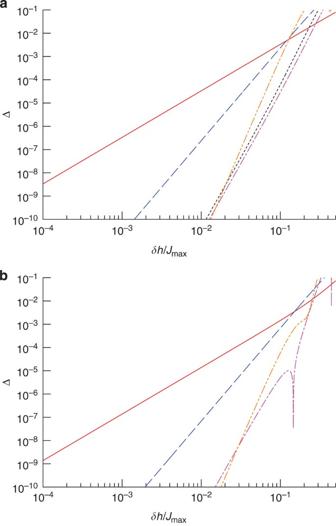Figure 3: Average error per gate for SUPCODE pulses ath0=0. These figures show the average error per gate Δ as functions ofδh/Jmaxfor the rotation around thezaxis by (a)φ0=π/2 and (b)φ0=1.7π. The red solid curves are for the uncorrected pulse with quadratic leading order errors inδh. Other curves are showing the three-piece (blue dashed lines), five-piece (black dotted line), seven-piece (magenta dash-dotted lines), and nine-piece (orange dash-dotted lines) SUPCODE pulses that cancel gate error Δ up through second, fourth, fourth and sixth order inδh, respectively. Figure 3: Average error per gate for SUPCODE pulses at h 0 =0. These figures show the average error per gate Δ as functions of δh / J max for the rotation around the z axis by ( a ) φ 0 = π /2 and ( b ) φ 0 =1.7 π . The red solid curves are for the uncorrected pulse with quadratic leading order errors in δh . Other curves are showing the three-piece (blue dashed lines), five-piece (black dotted line), seven-piece (magenta dash-dotted lines), and nine-piece (orange dash-dotted lines) SUPCODE pulses that cancel gate error Δ up through second, fourth, fourth and sixth order in δh , respectively. Full size image SUPCODE for h 0 ~ J max For h 0 ~ J max , the noncommutation of the Hamiltonian at different times even for δh =0 makes the previous approach algebraically forbidding. However, in this case, we have the possibility to perform rotations about axes other than . We make use of this freedom to construct SUPCODE pulses in a simple way: We first take an uncorrected (that is, designed as if δh =0) rotation and then construct an uncorrected identity operation designed such that the error in its implementation exactly cancels the leading order error in the original rotation. We represent the uncorrected rotations in terms of ideal rotations as and where and are the first order corrections. For the corrected pulse , it is clear that we want to make . Because there are infinitely many ways to realize the identity operation, there is sufficient freedom to engineer such a cancellation. In particular, we consider parameterized versions of the identity implemented as nested interrupted 2 nπ rotations about different axes, with two simple examples being and where a i and b i are parameters satisfying 0≤ a i ≤2π, 0≤ b i ≤ J max / h 0 and n is a positive integer. As an explicit demonstration of SUPCODE, we show rotations around the x and z axes by arbitrary angles 0< φ < π for the particular case J max / h 0 ≥5. (Combinations of these are sufficient for universal one-qubit gates.) About , the uncorrected rotation is performed by holding J =0 for a time φ / h 0 , and this is preceded by the identity where b 1 and b 2 are chosen such that errors cancel (see Methods as well as Supplementary Movie 2 ). About , the uncorrected rotation is performed by a three-part pulse [29] , [30] , and this is preceded by the identity where a , b 3 , and b 4 are chosen such that errors cancel (see Methods ). As shown in Fig. 4 for φ = π /2, SUPCODE does indeed lead to a higher order scaling of the error in δh / h 0 (and hence in ), and a reduction of error when δh / h 0 is less than a few percent. For instance, when δh / h 0 =5%, errors are typically reduced by an order of magnitude. 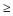Figure 4: Average error per gate for SUPCODE pulse atJmax/h05. This set of figures shows the average error per gate Δ as functions ofδh/h0, for rotations byπ/2 about the (a)xaxis and (b)zaxis. The red curves show the error per gate corresponding to the uncorrected pulses. The corrected pulses, shown by the blue dashed lines, cancel the leading order error. In this figure we usedh0as the energy scale instead ofJmax. Figure 4: Average error per gate for SUPCODE pulse at J max / h 0 5. This set of figures shows the average error per gate Δ as functions of δh / h 0 , for rotations by π /2 about the ( a ) x axis and ( b ) z axis. The red curves show the error per gate corresponding to the uncorrected pulses. The corrected pulses, shown by the blue dashed lines, cancel the leading order error. In this figure we used h 0 as the energy scale instead of J max . Full size image The tradeoff of our approach is that SUPCODE rotations are typically over an order of magnitude longer than uncorrected rotations. We note that for a given experimental set of parameters one should try optimizing the pulse sequence, which we have not done for the arbitrarily chosen example above, as both the length and error of the corrected pulses could certainly be reduced by a significant constant factor by searching over different constructions of the identity, Ĩ . Nonetheless, for experiments in GaAs systems with pumped nuclear spins [31] ( h 0 ~0.6 μeV, δh ~30 neV) or micromagnets [10] ( h 0 ~20 neV, δh ~1 neV), the sequences shown here could already deliver substantial improvement over the uncorrected ones. Realistic deviations from the ideal pulses assumed above would include charge noise, which adds a random quasi-static contribution to the exchange, and finite rise times. The former could be reduced by using a multi-electron variant of the singlet–triplet qubit [32] and, in principle, it may even be possible to dynamically correct by adding more degrees of freedom to the pulses. The latter can be compensated for by adjusting pulse parameters given the actual turn-on/off profiles of the pulse for a specific experimental set-up (we give explicit demonstrations in the Supplementary Discussion ). Thus, even in nonideal conditions SUPCODE could enable precise spin qubit rotations independent of shot-to-shot variation in the nuclear Overhauser field, also easing tasks such as ensemble-averaged measurements of singlet probability oscillations versus time by reducing hyperfine-induced decay. More importantly, this work allows satisfaction of the quantum error correction threshold within a substantially larger region of the physical parameter space than would otherwise be possible. The fact that T 2 has now reached tens of microseconds in GaAs quantum dots [7] , and milliseconds [18] or even seconds in the presence of isotopic purification [33] in Si-based structures implies that gate errors are currently dominated not by dynamical fluctuations in the nuclear spin bath, but by the statistical distribution of the magnetic field gradient, and these errors may be efficiently suppressed by SUPCODE. Expansion of the evolution operator around h 0 =0 The evolution operator is defined as with h = h 0 + δh . Expanding the evolution operator in powers of δh in the vicinity of h 0 =0, where one can show that and, for n >0, (note that the product is in descending order in observance of the time-ordering of operators) where and I is the 2×2 identity matrix and σ x , σ y , and σ z are Pauli matrices. Thus, for the n th-order term to vanish, one must have The no-go theorem shown in Supplementary Discussion implies that it is instructive to design pulses that cancel successive orders. In this work, we focus on the piecewise constant pulse, which can be expressed as where we have defined the dimensionless quantity τ k = J max t k for convenience, and t k refers to the duration of a pulse on the k th piece. The total duration of time after the k th piece would be , with T 0 ≡0 and T N ≡ T f indicating the initial and final time. J ( t ) can then be expressed as where Θ( t ) is the Heaviside step function. Three-piece SUPCODE for h 0 =0 Our motivation is to cancel successive orders of δh in the expansion with number of pieces N as small as possible. We consider symmetric pulses, that is, J ( t )= J ( T f − t ), for the h 0 =0 case. This ensures that U ( T f ,0) has no σ y component. [To see this fact, note that the operator can be written in the form A i = a i 0 I + a ix σ x + a iz σ z with a i 0 , a ix , a iz arbitrary complex numbers. It is then straightforward to show that for any operators A 1 and A 2 with arbitrary coefficients, A 2 · A 1 · A 2 can also be written in such a form, free of σ y terms. Applying this statement recursively to equation (15), one sees that for any J ( t ) satisfying J ( t )= J ( T f − t ) the resulting evolution operator U does not contain σ y component.] One of the simplest ways to cancel the leading order error with strictly positive values of J is via a three-piece pulse sequence. In equation (15), we take N =3 and the three-piece pulse sequence can be characterized by where φ 0 is the desired rotation angle around the z axis. It is straightforward to verify that the evolution operator under this pulse is Here the deviation from the desired rotation has been suppressed up to second order in δh (which corresponds to the fourth order in equation (2)). This pulse actually sweeps the Bloch vector through an angle φ =2 π + φ 0 , which is the origin of the trivial additional phase factor. It is clear that to achieve error cancellation, the Bloch vector generally must be swept through more than 2 π about the z axis as its path is deflected from the ideal ( δh =0) path in opposite directions in the 'eastern and western hemispheres'. (One can also explicitly show the necessity of larger angles from equation (10).) Thus the three-piece pulse sequence cancels leading order error simply by ensuring that, in the absence of δh , the Bloch vector spends an equal amount of time in each hemisphere during its rotation. Five-piece SUPCODE for h 0 =0 We set N =5 in equation (15), which allows us to cancel the dependence of U ( T f ,0) on δh up to the second order (corresponding to the fourth order in equation (2)), using a symmetric pulse with parameters J 1 = J 3 = J 5 =0, J 2 = J 4 = J max , and We expand U ( T f ,0) as To make the first order coefficient vanish, one must choose Plugging equation (21) into equation (20), it suffices to satisfy to make the second order terms vanish. We choose a root that is positive for 2 π <φ<3π, that is Equations (19), (21), and (23) prescribe the pulse parameters required to achieve a rotation while cancelling the dependence of U ( T f ,0) on δh up to the second order. A plot of these parameters as a function of φ is given in Fig. 1 . This pulse is defined for , which is equivalent to a rotation with . Rotation of angles outside the range (0, π ) may be achieved by duplicating existing pulse sequences. For example, to achieve a rotation of φ 0 =1.2 π , one could apply twice the φ 0 =0.6 π (corresponding to φ =2.6 π ) rotation. As φ →2 π , τ 1 →∞, τ 2 = π /2, τ 3 →2 τ 1 . If we want to fix the total duration of the sequence, we let J max →∞. The pulse sequence becomes the well-known CPMG pulse [13] , [14] . In fact, it can be shown that for a pair of instantaneous π pulses, setting leading order errors to zero while maintaining the time-reversal symmetry of the pulse sequence enforces the Uhrig condition [15] . For details of the construction of seven-piece and nine-piece SUPCODE, see Supplementary Methods . SUPCODE for h 0 ≠0 As described in Results, we perform corrected rotations as where the implementation of the identity Ĩ is chosen such that the first order errors in δh exactly cancel those from the rotation . Our implementations of Ĩ are of the form For the specific forms Ĩ 1 , Ĩ 2 given in the main text, the parameters a i , b i are constrained by The particular implementation of Ĩ that will be chosen for a given experimental situation will depend on the particular rotation as well as the experimental parameters J max / h 0 , with a combinatorial search necessary to find an implementation that (a) cancels the first-order error from ; (b) satisfies the constraints of equations (25) and (26); and (c) is close to 'optimal' in some experimentally meaningful sense, such as having the overall shortest duration in time, having the smallest second-order error in δh , or being least sensitive to over-/under-shoot in J ( t ). As an example of our technique, we found sequences valid for the experimentally relevant regime J max / h 0 ≥5, for corrected rotations about angles 0≤φ≤ π around the x and z axes. (We have also verified that slightly more complicated identities can be constructed to correct error for pulses with smaller values of J max / h 0 >1.5.) For the x axis rotation, we have The first-order term in δh is zero when b 1,2 are chosen to satisfy The solution to these equations are shown in Supplementary Fig. S1 . In Supplementary Fig. S1a, we show a specific example of the pulse sequence for π /2 rotation about the x axis, and correspondingly, we show how a given state evolves under this SUPCODE in Supplementary Movie 2 . Supplementary Fig. S1c shows solutions for a range of rotation angle 0≤ φ ≤ π . For the same parameter range, we construct the corrected z axis rotation as with a and b3,4 satisfying The solution to these equations is shown in Supplementary Fig. S2 . In Supplementary Fig. S2a, we show an example of the pulse sequence appropriate for rotating about the z axis by π /2, while in Supplementary Fig. S2c, we show solutions for 0≤φ≤π. How to cite this article: Wang X. et al . Composite pulses for robust universal control of singlet–triplet qubits. Nat. Commun. 3:997 doi: 10.1038/ncomms2003 (2012).